Cooperative chalcogen bonding interactions in confined sites activate aziridines 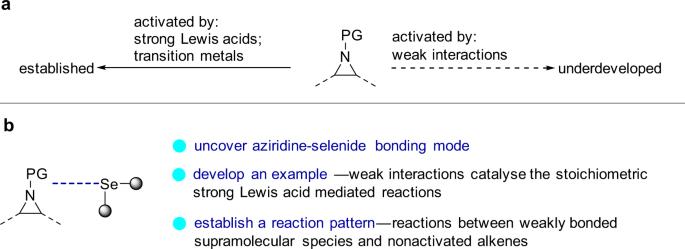Fig. 1: Distinct approaches to the activation of aziridines. aActivation of aziridines: the state of the art.bThis work: chalcogen bonding activation and catalysis approach. The activation of aziridines typically involves the use of strong Lewis acids or transition metals, and methods relying on weak interactions are rare. Herein, we report that cooperative chalcogen bonding interactions in confined sites can activate sulfonyl-protected aziridines. Among the several possible distinct bonding modes, our experiments and computational studies suggest that an activation mode involving the cooperative Se···O and Se···N interactions is in operation. The catalytic reactions between weakly bonded supramolecular species and nonactivated alkenes are considered as unfavorable approaches. However, here we show that the activation of aziridines by cooperative Se···O and Se···N interactions enables the cycloaddition of weakly bonded aziridine-selenide complex with nonactivated alkenes in a catalytic manner. Thus, weak interactions can indeed enable these transformations and are an alternative to methods relying on strong Lewis acids. Weak interactions are among the significant evolutionary forces that are smartly exploited by nature to modulate the conformation of proteins and to drive cellular reactions. The simulation of this biomimetic strategy in supramolecular catalysis has gained fruitful achievements in promoting chemical reactions [1] , [2] , [3] , [4] , [5] , [6] , [7] , [8] , [9] , [10] . Amongst these interactions, catalysis with hydrogen bond plays a dominant role while halogen [2] , [3] , [4] , as well as chalcogen bonding catalysis [5] , [6] , [7] , [8] , [9] , has lately attracted ever-increasing research interest. Since the weak interactions restrict both the reactivity and the concentration of equilibrating supramolecular complex, this catalysis discipline has its constraint boundary considering the limitations of the activation targets and reaction patterns [10] . Even though weak interactions can activate a range of molecules such as carbonyl compounds, imines, nitro olefins, etc., it is a challenging task for these interactions to activate target molecules like aziridines which were conventionally handled by strong Lewis acids or transition metals. (Fig. 1a ) [10] . Furthermore, the reactants suitable for trapping these weakly bonded supramolecular species have specific requirements, thus partly restricting the reaction patterns. For instance, the reactions between weakly bonded supramolecular species and nonactivated alkenes are considered unfavorable approaches in supramolecular catalysis [10] . To develop this field, research toward expanding the activation targets and establishing distinct reaction patterns is of vital importance. Fig. 1: Distinct approaches to the activation of aziridines. a Activation of aziridines: the state of the art. b This work: chalcogen bonding activation and catalysis approach. Full size image Chalcogen bonding [11] , the noncovalent interaction between an electron donor and a chalcogen atom incorporated in a specific molecular entity, has recently found application in drug design [12] , material chemistry [13] , intramolecularly conformational control [14] , [15] , [16] , [17] , [18] , anion recognition and transport processes [19] , [20] , [21] , [22] , [23] , [24] , [25] , [26] . The theoretical investigation suggests that charge transfer, disperse force, and electrostatic potential are significant contributors to the formation of chalcogen bonding interactions [6] . As the chalcogen bond, in general, is weak [27] , catalysis with chalcogen bonding interactions based on divalent chalcoether is thus a rarely explored concept and a limited number of examples were introduced [28] , [29] , [30] , [31] , [32] , [33] , [34] , [35] , [36] , [37] . Herein, we report the chalcogen bonding mode of the aziridine-selenide complex and the catalytic reactions between these supramolecular complexes and nonactivated alkenes. We show that weak interactions enable catalytic transformations, in contrast with methods relying on stoichiometric strong Lewis acid-mediated organic transformations (Fig. 1b ). Bonding property We recently developed a class of phosphonium selenide-based chalcogen bonding catalysts, which showed catalytic activity in the activation of carbonyl groups and vinylindoles [28] , [29] , [30] , [31] . Since there are multiple Lewis basic sites in sulfonyl-protected aziridine like 1a / 1a ′ (Fig. 2a ), the binding modes for activating aziridines with such phosphonium selenides are much more complicated and the interactions with proper sites are crucial to the generation of catalytic capability. To understand the distinct bonding behavior of monodentate and bidentate chalcogen bonding donors Ch1 - 6 with sulfonyl-protected aziridine, 77 Se NMR analysis of the bonding complexes was carried out (Fig. 2 ). Upon using monodentate chalcogen bonding donors Ch1-2 associated with \({{{{{\mathrm{GaCl}}}}}}_{4}^{-}\) or a less coordinating counteranion, i.e. \({{{{{\mathrm{BAr}}}}}}^{{{{{\mathrm{F}}}}}}_{{4}^{-}}\) (tetrakis(3,5-bis(trifluoromethyl)phenyl)borate), analysis of the mixture of Ch1 / 2 and aziridine 1a by 77 Se NMR showed that the chemical shift of the 77 Se signal almost remains unchanged even in the presence of 9.0 equivalent of aziridine 1a (Fig. 2a ). These observations suggest that a single chalcogen bonding interaction between Ch1 / 2 and aziridine gives short-life supramolecular species with very low concentration. Fig. 2: Chalcogen bonding interactions between Ch1-6 and aziridines ( 77 Se NMR in CD 2 Cl 2 , 76 MHz, and 298 K). a Chalcogen bonding between monodentate catalysts Ch1 - 2 and aziridine 1a . b Chalcogen bonding between bidentate catalysts Ch3 - 6 and aziridine 1a/1a ′. Full size image Upon forming intermolecular interaction with 1a / 1a ′, the distinct structure of Ch3-6 leads to the variation of the 77 Se signal in a different extent (Fig. 2b ). Analysis of the mixture of Ch3 and 1a by 77 Se NMR reveals that the chemical shift of the 77 Se signal varies by 0.34 ppm while the 31 P signal almost remains unchanged (<0.05 ppm), indicating that the interaction between selenium and aziridine induces the change of the 77 Se signal. The interaction of Ch4 with 1a also resulted in an observable variation of the 77 Se signal (0.11 ppm). In sharp contrast, an as much as 1.23 ppm down-filed shift of the 77 Se signal was observed in the presence of Ch6 . Since 1a was not stable enough in the presence of Ch5 , the variation of 77 Se signal, in this case, is invalid. Further investigation using aziridine 1b shows a similar trend of perturbation and the interaction of Ch6 and 1b gave the most dramatic change in the 77 Se signal. These observations pose a confusing phenomenon that the variation of the 77 Se signals of Ch5 and Ch6 is much more dramatic than chalcogen bonding donors Ch3 and Ch4 . To explain the aforementioned observations, the relationship between bonding and structure was investigated (Fig. 3a ). To this end, the crystal structures of catalysts Ch3 , Ch5 , and Ch6 associated with a \({{{{{\mathrm{BAr}}}}}}^{{{{{\mathrm{F}}}}}}_{{4}^{-}}\) counteranion were obtained. The crystal data for Ch4 associated with \({{{{{\mathrm{BAr}}}}}}^{{{{{\mathrm{F}}}}}}_{{4}^{-}}\) was obtained previously [31] and it would provide insightful information to elucidate its structure herein. The intramolecular chalcogen bonding interactions were observed in the crystal structures Ch3 - 5 (Fig. 3a ). These weak interactions are in agreement with the properties of chalcogen bonding since the separation between the two contact atoms is shorter than the sum of their van der Waals radii while the electron donor approaches the selenium atom approximately along the direction of the axis of C‒Se covalent bond [10] . The crystal structure of Ch3 shows two Se···O bonding interactions while its rigid counterpart Ch4 shows the presence of a ‘like-like’ Se···Se interaction and a Se···O interaction between the two bonding units. The bonding behavior of Ch3 is similar to the previously observed structure of Ch4 associated with a TfO ‒ counteranion [29] , which also shows two intramolecular Se···O bonding interactions. These observations indicate the counteranion can pronouncedly affect the bonding interactions. The crystal structure of Ch5 exhibits the Se···π bonding interactions between the selenium in one unit and the phenyl ring in the other unit. In contrast, no intramolecular chalcogen bonding interaction was observed in the crystal structure of Ch6 . While X-ray crystallographic data of Ch5 and Ch6 indicate solvent in the crystals, powder X-ray diffraction (PXRD) data of Ch3 - 6 are in agreement with the simulated results from corresponding single crystal diffraction data (see Supplementary Figs. 28 – 31 ). Fig. 3: Relationship between bonding and structure. a X-ray crystal structures of Ch3 - 6 (hydrogens and counteranions were omitted for clarity; the selenium atoms are disordered and no chalcogen bonding interaction in Ch6 ). b Equilibrium between intramolecular chalcogen bonding and non-bonding status of catalysts Ch3 - 5 and catalyst Ch6 . Full size image Owing to the presence of the intramolecular Se···O interaction in Ch3 as well as both Se···O and Se···Se interactions in Ch4 (Fig. 3b ), the addition of aziridine 1a / 1a ′ competitively generates the intermolecular Se···O and Se···N interactions which are the similar type relative to the intramolecular interactions, thus resulting in less variation of the 77 Se signals as shown in Fig. 2 . In contrast, in the case of Ch5 or Ch6 which does not have an intramolecular Se···O or Se···Se interaction, the intermolecular Se···O and Se···N interactions with 1a / 1a ′ would substantially change the bonding status of Ch5 and Ch6 , thus inducing more marked variation of the 77 Se signals. Bonding mode To investigate the active bonding modes (Fig. 4a ), a range of molecular control experiments were carried out as depicted in Fig. 4b–e (see Supplementary Figs. 7 – 22 ). Using aziridine m1 a model Lewis base, the control 13 C NMR experiments reveal that the chemical shift of C α (attached to S) almost remains unchanged while the chemical shift of the more remote C β (two bonds from S) varies dramatically when comparing the bonding performance of monodentate catalyst Ch2 ( Ch2 : m1 2:1) and their counterparts, bidentate catalysts Ch5 and Ch6 ( Ch : m1 1:1) (Fig. 4b ). For a bidentate catalyst, it is unlikely that the shifting from a single interaction mode (i.e., SC0 or SC1 ) to a mode of double interaction with oxygen (i.e., SC4 or SC5) would lead to almost no perturbation of the chemical shift of C α while resulting in a marked variation of C β . Instead, the dramatic change of C β attached to nitrogen indicates that a double interaction mode involving the direct interaction with nitrogen (i.e., SC6 ) is a reasonable binding mode to explain the experimental results. For a much sharper contrast, the formation of the complexes between Ch5 / 6 and m1 led to a negligible variation of C α (0.07 and 0.06 ppm) while resulting in a much more pronounced change of C β (0.65 and 0.55 ppm), which also suggests the direct interaction with nitrogen (i.e., SC6 ) to be the active complex. To give a more direct comparison, twofold Ch7 ( Ch7 : m1 2:1) was used, i.e., monodentate version of Ch5 and Ch6 , and similar results were obtained. Further using m2 as a model Lewis base gave similar observations. Fig. 4: Probing binding modes ( 13 C NMR in CD 2 Cl 2 , 100 MHz, 298 K). a Distinct binding modes. b Comparable chalcogen bonding experiments between monodentate and bidentate catalysts. c Comparable chalcogen bonding experiments between aziridine and its ring-opening counterpart. d Comparable chalcogen bonding experiments between catalysts Ch4 - 6 and m4 - 5 . 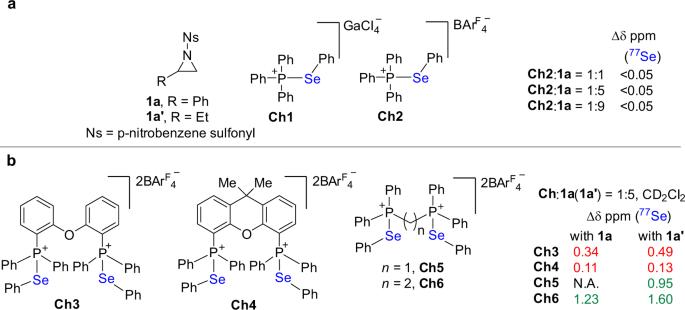Fig. 2: Chalcogen bonding interactions between Ch1-6 and aziridines (77Se NMR in CD2Cl2, 76 MHz, and 298 K). aChalcogen bonding between monodentate catalystsCh1-2and aziridine1a.bChalcogen bonding between bidentate catalystsCh3-6and aziridine1a/1a′. e Substitution group effect on chalcogen bonding between aziridines m6 - 7 and catalysts Ch4 - 6 . Full size image The subsequent molecular control experiments further support SC6 as the active binding species. As shown in Fig. 4c , in contrast to aziridine 1a ′, its ring-opening counterpart m3 almost gave no change in the chemical shift of C β regardless of in the presence of a monodentate or a bidentate catalyst. These observations indicate the structure of the nitrogen part is critically important to the chalcogen bonding interactions. The distinct perturbation of the chemical shift of C β between aziridine 1a ′ and its ring-opening counterpart m3 suggests a direct interaction with nitrogen (i.e., SC6 ) is in operation rather than interaction with the relatively more remote oxygen ( SC4 or SC5 ). The results of the molecular balance experiments in Fig. 4d are further against a double interaction mode with oxygen (i.e., SC4 and SC5 ). For C β in the piperidine ring, the variation of the chemical shift decreased from m4 to m5 . However, a reverse variation of C β′ relative to C β was observed, that is, a decreased variation of the chemical shift of C β leads to an increased variation of the chemical shift of C β′ . These molecular balance experiments indicate the equilibrating interaction with one of the two nitrogen parts is more favorable, thus suggesting binding modes SC6 is operative rather than SC4 or SC5 . Further investigation reveals that the substitution group in the aziridine ring has a pronounced effect on the variation of the chemical shift of the ring carbons attached to nitrogen (Fig. 4e ). It was found that the ring carbon C β in m6 with an aliphatic substitution (i.e., Me) resulted in a marked variation of the chemical shift while the ring carbon C β in m7 with an aromatic substitution (i.e., Ph) almost remains unchanged ( Ch4 ) or even shifted to a reverse direction ( Ch5 , Ch6 ). These experiments indicate the substitution group in the aziridine ring can largely affect the interactions, thus pointing out a mode involving the direct interaction with the nitrogen atom (i.e., SC6 ). Therefore, the molecular control experiments depicted in Fig. 4b–e suggest SC6 is the active binding mode of bidentate chalcogen bonding donors Ch4 - 6 . The binding mode of SC6 between Ch5 and 1-(phenylsulfonyl)aziridine were further corroborated by DFT calculations (see Supplementary Tables 5 – 7 ). The complexes were optimized at the M06-2X/6-31 g(d,p) level of theory corrected with Grimme’s dispersion (D3) [38] . The optimized structure of SC6 (Fig. 5a ) shows the simultaneously cooperative Se···O and Se···N interactions confirmed by QTAIM analyses with interaction energy of −23.7 kcal/mol, while the complex SC3 with a single Se···N interaction has weaker interaction energy of −20.6 kcal/mol. The relative Gibbs free energy for SC6 is −8.3 kcal/mol which is lower than that of SC3 (−5.9 kcal/mol), suggesting that the formation of SC6 is more favorable and feasible. These calculated energies are in a reasonable range considering the literature precedents [32] , [39] . Natural bond orbital (NBO) analyses of SC3 and SC6 (Fig. 5b ) further suggest that the Se···N interaction between Ch5 and aziridine in SC3 plays a significant role. In contrast, both the Se···O and Se···N interactions between Ch5 and aziridine in SC6 play important roles. Fig. 5: DFT calculations. a The optimized structures of the complexes SC3 and SC6 between Ch5 and 1-(phenylsulfonyl)aziridine. b The key intermolecular donor-acceptor orbital interactions between Ch5 and 1-(phenylsulfonyl)aziridine in SC3 (I) and SC6 (II-IV); BD*(1) denotes the σ* antibonding orbital; LP(1) and LP(3) denote the first and third lone-pair orbitals, respectively. Full size image Chalcogen bonding catalysis The reactions between weakly bonded supramolecular species and nonactivated alkenes are considered unfavorable transformations [1] , [2] , [3] , [4] , [5] , [6] , [7] , [8] , [9] , [10] . Therefore, to apply the bonding property of the aziridine-selenide complex, the cycloaddition of aziridines with nonactivated alkenes was selected as a target reaction as literature reports indicate that it would be a tough challenge for a weak interaction to promote this reaction (Fig. 6 ) [40] , [41] , [42] , [43] . To generate reactivity, the reported precedent used strong Lewis acid BF 3 ·OEt 2 to promote this reaction (Fig. 6a ) [40] , [41] . Moreover, in order to generate a proper concentration of intermediate suitable for trapping with nonactivated alkenes, a stoichiometric amount of BF 3 ·OEt 2 was used. Otherwise, the reaction has to be carried out under a thermal-driven condition (100 °C) to give reactivity in the presence of a transition-metal catalyst [42] , [43] . To achieve this reaction by a weak interaction, there are two challenging problems (Fig. 6b ). As the weak interaction provides much less activation than the strong Lewis acid counterpart, one problem is thus how a weak interaction with aziridine can give rise to activation ability. Furthermore, in contrast to the strong Lewis acid counterpart, the weak interaction always results in the generation of an unstable supramolecular complex with low concentration. Therefore, the other glaring problem is how to increase the concentration of aziridine-mediated supramolecular species to a reactive level by only using a catalytic amount of noncovalent activator. In this context, the chalcogen bonding approach was applied to address these problems. Fig. 6: Shifting stoichiometric strong Lewis acid approach to chalcogen bonding catalysis. a Stoichiometric strong Lewis acid approach. b A challenging proposal: catalysis by weak interactions. Full size image Initially, to evaluate the reactivity of this cycloaddition process towards activation by noncovalent interactions, the well-established hydrogen-bonding donors H1 - 3 were employed as references (Fig. 7a ). There was no background reaction even after 24 h in the absence of a catalyst. In the presence of 10 mol % of a typical hydrogen-bonding donor ( H1 - 3 ), the reaction did not work. Furthermore, only a trace amount of product 3a (<5%) was obtained using a stoichiometric amount of a hydrogen-bonding catalyst H1 (1.0 equiv), indicating inertness of this reaction under activation by weak interactions. Considering the poor reactivity of this cycloaddition reaction, we envisioned that cooperative chalcogen–bonding interactions with aziridine would enhance the activation ability and provide more stabilization of the supramolecular species, thus improving the reactivity. However, to match the confined Lewis basic binding sites in phenylsulfonyl protected aziridines, the judicious use of bidentate chalcogen bonding donors that are capable of precisely recognizing the proper Lewis basic sites of aziridine is critically important to give catalytic activity (Fig. 7b ). Fig. 7: Noncovalent catalysis approach to cycloaddition of aziridine 1a with nonactivated alkene 2a. a Catalysis with typical hydrogen-bonding donors. b The interactions between bidentate chalcogen bonding donors and phenylsulfonyl protected aziridines. c Chalcogen bonding catalysis approach to cycloaddition of aziridines with nonactivated alkenes. d Inhibition experiment. DCE 1, 2-dichloroethane. Full size image In consistence with the results in Figs. 2 , 4 , upon using monodentate chalcogen bonding donors Ch1 - 2 as catalysts, the reaction did not work. Nonetheless, these experiments revealed that neither the phosphonium unit nor the BAr F 4 ˉ counterion is catalytically active (Fig. 7c ). To implement the idea as depicted in Fig. 7b , two sets of bidentate catalysts were investigated. One set is catalyst Ch3 with a free rotation linker and its rigidified counterpart Ch4 . The other set is catalysts Ch5 - 7 with different lengths of linkers. The comprehensive control experiments (see Supplementary Figs. 15 – 22 ) indicate Ch3 bearing a long linker with free rotation between two chalcogen bonding sites operates like a monodentate catalyst. In consistence with these observations, the experimental results revealed that catalyst Ch3 with a long and free rotation linker gave no catalytic activity. Then the free rotation linker of catalyst Ch3 was rigidified. Upon changing catalyst Ch3 to catalyst Ch4 with a rigid backbone, the reaction began to work and catalyst Ch4 showed high catalytic activity to give a 77% yield of product 3a at room temperature. Analysis of the mixture of Ch4 and olefin 2a by 77 Se and 31 P NMR indicated that there was no detectable variation of the 77 Se and 31 P signals, indicating there is no competitive bonding between catalysts Ch4 and 2a (see Supplementary Fig. 23 ). Further investigation of the catalytic performance of the bidentate catalysts Ch5 - 6 suggests the distance between the two binding sites is critically important. Upon linking the two phosphonium units with one carbon, catalyst Ch5 exhibited good catalytic activity to give a 75% yield of 3a , indicating this distance between the two binding sites can well interact with the proper Lewis basic sites of aziridine. In contrast to Ch5 , even only increasing the length of the linker by one carbon, catalyst Ch6 showed poor catalytic activity and only a 13% yield of 3a was obtained. In contrast, monodentate catalyst Ch7 had no catalytic activity. Similar to the case of Ch3 , upon linking the two phosphonium units with five carbons, catalyst Ch8 with improperly positioned two binding sites completely lost catalytic activity. Catalyst Ch9 with electron-withdrawing substituents on the aryl ring did not show catalytic activity. For the same selenide, the strength of chalcogen bonding interaction is determined by the electron-donating ability of aziridines. Therefore, toluenesulfonyl-protected aziridine in principle generates stronger chalcogen bonding interactions than nitrobenzenesulfonyl-protected aziridine. 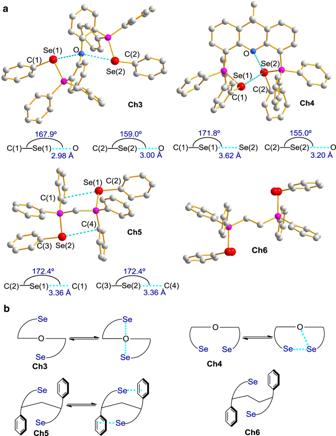Fig. 3: Relationship between bonding and structure. aX-ray crystal structures ofCh3-6(hydrogens and counteranions were omitted for clarity; the selenium atoms are disordered and no chalcogen bonding interaction inCh6).bEquilibrium between intramolecular chalcogen bonding and non-bonding status of catalystsCh3-5and catalystCh6. In line with this notion, analysis of a mixture of N -( p -toluenesulfonyl)aziridine ( 1b , i.e., Ns in 1a was replaced by Ts) and 10 mol% selenide Ch5 in DCE by TLC revealed that 1b was fully decomposed after only 80 s at room temperature, which was further supported by 1 H NMR analysis of this mixture. In sharp contrast, for a reaction mixture of N -( p -nitrobenzenesulfonyl)aziridine 1a and 10 mol% selenide Ch5 in DCE, 76% 1a remained unchanged after 80 s. To corroborate these observations, further analysis of a 1:1 competitive mixture of 1a and 1b in the presence of 10 mol% selenide Ch5 in CD 2 Cl 2 indicated that 1b was fully decomposed while 81% of 1a remained unchanged in this reaction mixture after 80 s. Therefore, in order to suppress side reaction pathways, nitrobenzenesulfonyl protecting group is an optimal choice. Since the weak nature of chalcogen bonding interactions restricts both the reactivity and the concentration of equilibrating aziridine-selenide complex, the control experiment (Fig. 7d ) demonstrate that only the addition of 1 mol% tetrahydrothiopyran almost resulted in complete inhibition of the reaction even in the presence of 10 mol% catalyst Ch4 (<5% 3a ). In line with the analysis as depicted in Fig. 6b , this experiment suggests that only a very low concentration of complex SC6 was generated and it is susceptible to completive bonding. While the experiments in Fig. 4 indicate catalyst Ch6 could act as an effective bidentate chalcogen bonding donor to form complex SC6 , however, Ch6 is less efficient to activate electron-deficient Ns-protected aziridines in contrast to its counterpart Ch4 or Ch5 . On the other hand, comparable results on the interactions of more electron-rich aziridines m1 - 2 with Ch5 and Ch6 were observed (Fig. 4b ), indicating the interaction of Ch6 and aziridine is affected by the electronic effect of aziridines. Based on these observations, the contrast experiments on the catalytic performance of Ch6 in CH 2 Cl 2 using aziridines with different electronic properties were carried out (Fig. 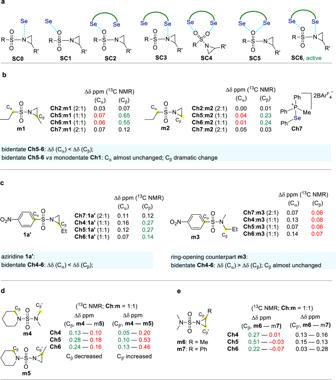Fig. 4: Probing binding modes (13C NMR in CD2Cl2, 100 MHz, 298 K). aDistinct binding modes.bComparable chalcogen bonding experiments between monodentate and bidentate catalysts.cComparable chalcogen bonding experiments between aziridine and its ring-opening counterpart.dComparable chalcogen bonding experiments between catalystsCh4-6andm4-5.eSubstitution group effect on chalcogen bonding between aziridinesm6-7and catalystsCh4-6. 8 ). The control experiments using p - t -BuPh, p -ClPh, and Ph substituted aziridines as substrates showed distinct results (yield: 52% for p - t -BuPh; 14% for Ph; 7% for p -ClPh). Fig. 8: Control experiments on the catalytic performance of Ch6 by using aziridines with different electronic properties. Reaction conditions: the reactions were carried out by using aziridine 1 (0.1 mmol), 2a (0.3 mmol, 25.2 mg), Ch6 (0.01 mmol, 10 mol %, 24.4 mg) in CH 2 Cl 2 (1.5 mL) at room temperature under argon for 12 h. Full size image As shown in Fig. 9a , the reaction time can be shortened from 10 to 1 h while the yield of product 3a was improved from 77 to 85% upon conducting the reaction at 50 °C. Tracing the reaction system by 31 P NMR reveals that catalyst Ch4 is stable in this reaction process and only the 31 P signal of catalyst Ch4 was observed (see Supplementary Fig. 2 ). Different protecting groups can be tolerated in this reaction to give products 3b and 3c in 60 and 67% yields, respectively. Terminal olefins with different chain length showed similar reactivity. A tetrasubstituted olefin was highly reactive to give pyrrolidine 3f in an 82% yield. Cycloalkyl-substituted olefins were used to give different spiro-pyrrolidines 3g – k in good yields. Regardless of the electronic characteristic of the substituents on the aromatic ring as well as the positions where the substitution groups are located, aziridines bearing different aromatic rings were well tolerated to give pyrrolidines 3l – u with reasonable yields. Mono-substituted nonactivated alkene was proven to be an effective reactant, and product 3v was obtained in 53% yield (dr: 3:1). Furthermore, alkynes were also effective substrates [44] , and products 5a - 5i were obtained in 60–79% yields (Fig. 9b ). Upon using ketones as substrates [44] , products 7a and 7b were obtained in 83 and 67% yields, respectively (Fig. 9c ). Fig. 9: Reaction scope. a Reactions between aziridines and alkenes. b Reactions between aziridines and alkynes. c Reactions between aziridines and ketones. Full size image In summary, this manuscript reports the chalcogen bonding of aziridine-selenide complexes and establishes a type of reaction between weakly bonded supramolecular species and nonactivated alkenes, thus shifting the stoichiometric strong Lewis acid-mediated approach to a noncovalent catalysis manner. Experimental results revealed that the bidentate catalysts with confined binding distance enable the simultaneous formation of Se∙∙∙O and Se∙∙∙N interactions with aziridines, which enables their use in catalysis. This research opens up opportunities for addressing problems relative to activation targets and reaction patterns in supramolecular catalysis. General procedure for the preparation of bidentate chalcogen bonding catalysts Ch3-6 and Ch8 To a red solution of PhSeCl (383.0 mg, 2.0 mmol) in dry Et 2 O (6.0 mL) at 0 °C under argon was added TMSOTf (444.5 mg, 2.0 mmol). The reaction mixture was allowed to warm up to room temperature and stirred for 40 min to give a dark orange solution. Then 1.0 mmol phosphine ([oxybis(2,1-phenylene)]bis(diphenylphosphine) for Ch3 ; (9,9-dimethyl-9H-xanthene-4,5-diyl)bis(diphenylphosphine) for Ch4 ; bis(diphenylphosphino)methane for Ch5 ; 1,2-bis(diphenylphosphino)ethane for Ch6 ; 1,5-bis(diphenylphosphino)pentane for Ch8 ) dissolved in dry CH 2 Cl 2 (4.0 mL) was added over 5 min at 0 °C. The reaction mixture was allowed to warm up to room temperature and stand for 1 h. The white solid suspension was filtered and washed by anhydrous diethyl ether. Then sodium tetrakis[3,5-bis(trifluoromethyl)phenyl]borate (1772.4 mg, 2.0 mmol) was added to a solution of the above white solid (1.0 mmol) in dry CH 2 Cl 2 (10.0 mL) under argon and the reaction mixture was stirred at room temperature for 24 h. Then the reaction mixture was filtered and the filtrate was concentrated to give a saturated solution under reduced pressure and then 10.0 mL n -hexane was slowly added. The two-phase solution was placed at room temperature under argon and the desired product precipitated out as a white solid. Then the precipitated white solid was collected by filtration and recrystallized twice from CH 2 Cl 2 (or ether) and n -hexane to afford the pure catalyst. General procedure for the preparation of monodentate chalcogen bonding catalysts Ch2, Ch7, and Ch9 To a red solution of PhSeCl (191.5 mg, 1.0 mmol for catalysts Ch2 and Ch7 ) or 3,5-F 2 C 6 H 3 SeCl (227.9 mg, 1.0 mmol for catalyst Ch9 ) in dry Et 2 O (6.0 mL) at 0 °C under argon was added TMSOTf (222.3 mg, 1.0 mmol). The reaction mixture was allowed to warm up to room temperature and stirred for 40 min to give a dark orange solution. Then 1.0 mmol phosphine (triphenylphosphine for Ch2 and Ch9 ; methyldiphenylphosphine for Ch7 ) dissolved in dry CH 2 Cl 2 (4.0 mL) was added over 5 min at 0 °C. 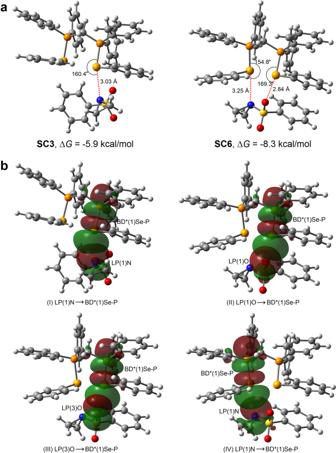Fig. 5: DFT calculations. aThe optimized structures of the complexesSC3andSC6betweenCh5and 1-(phenylsulfonyl)aziridine.bThe key intermolecular donor-acceptor orbital interactions betweenCh5and 1-(phenylsulfonyl)aziridine inSC3(I) andSC6(II-IV); BD*(1) denotes the σ* antibonding orbital; LP(1) and LP(3) denote the first and third lone-pair orbitals, respectively. The reaction mixture was allowed to warm up to room temperature and stand for 1 h. Then sodium tetrakis[3,5-bis(trifluoromethyl)phenyl]borate (886.2 mg, 1.0 mmol) was added to the above reaction system and stirred at room temperature for 24 h. Then the reaction mixture was filtered and the filtrate was concentrated to give a saturated solution under reduced pressure and then 10.0 mL n -hexane was slowly added. The two-phase solution was placed at room temperature under argon and the desirable product precipitated out as a white solid. Then the precipitated white solid was collected by filtration and recrystallized twice from CH 2 Cl 2 and n -hexane to afford the pure catalyst. General procedures for chalcogen bonding catalysis of cycloaddition reactions To a reaction mixture of aziridine 1 (0.2 mmol) and catalyst Ch4 (10 mol %, 52.4 mg, 0.02 mmol) in a 10-mL-Schlenk tube was added DCE (1.0 mL) under argon atmosphere. 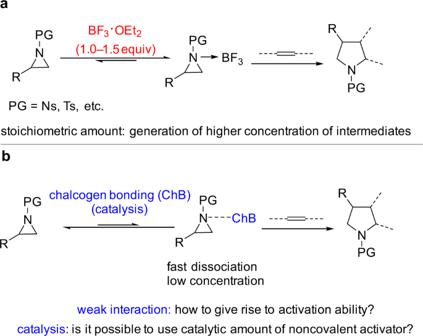Fig. 6: Shifting stoichiometric strong Lewis acid approach to chalcogen bonding catalysis. aStoichiometric strong Lewis acid approach.bA challenging proposal: catalysis by weak interactions. Then the corresponding reactant alkene 2 or alkyne 4 or ketone 6 (0.6 mmol, 3.0 equiv) was added to the above reaction mixture. The reaction was stirred at indicated temperature (50 °C for the reactions to generate products 3 and 7 ; room temperature for the reactions to generate product 5 ) until the completion of the reaction as judged by TLC analysis. 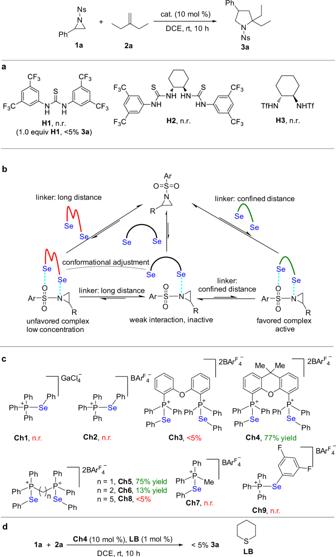Fig. 7: Noncovalent catalysis approach to cycloaddition of aziridine 1a with nonactivated alkene 2a. aCatalysis with typical hydrogen-bonding donors.bThe interactions between bidentate chalcogen bonding donors and phenylsulfonyl protected aziridines.cChalcogen bonding catalysis approach to cycloaddition of aziridines with nonactivated alkenes.dInhibition experiment. DCE 1, 2-dichloroethane. 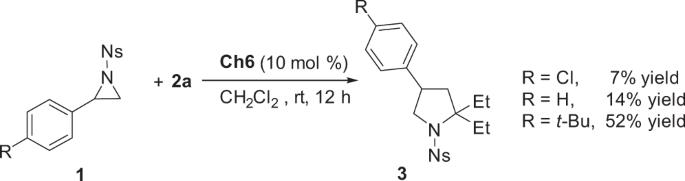Fig. 8: Control experiments on the catalytic performance of Ch6 by using aziridines with different electronic properties. Reaction conditions: the reactions were carried out by using aziridine1(0.1 mmol),2a(0.3 mmol, 25.2 mg),Ch6(0.01 mmol, 10 mol %, 24.4 mg) in CH2Cl2(1.5 mL) at room temperature under argon for 12 h. 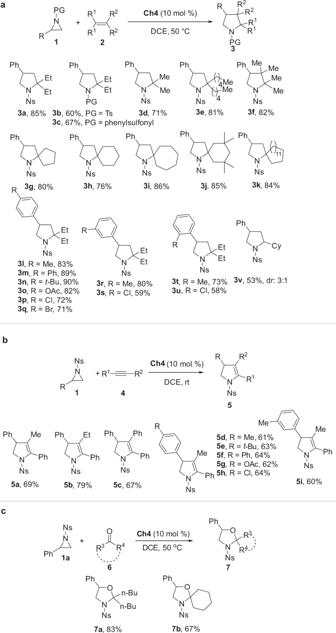Fig. 9: Reaction scope. aReactions between aziridines and alkenes.bReactions between aziridines and alkynes.cReactions between aziridines and ketones. Then the solvent was removed under reduced pressure and the residue was purified by flash chromatography on silica gel using petroleum ether/ethyl acetate (v/v = 30:1 to 10:1) as eluent to give the desired products.